A subunit-selective potentiator of NR2C- and NR2D-containing NMDA receptors NMDA receptors are tetrameric complexes of NR1 and NR2A–D subunits that mediate excitatory synaptic transmission and have a role in neurological disorders. In this article, we identify a novel subunit-selective potentiator of NMDA receptors containing the NR2C or NR2D subunit, which could allow selective modification of circuit function in regions expressing NR2C/D subunits. The substituted tetrahydroisoquinoline CIQ (3-chlorophenyl)(6,7-dimethoxy-1-((4-methoxyphenoxy)methyl)-3,4-dihydroisoquinolin-2(1 H)-yl)methanone) enhances receptor responses two-fold with an EC 50 of 3 μM by increasing channel opening frequency without altering mean open time or EC 50 values for glutamate or glycine. The actions of CIQ depend on a single residue in the M1 region (NR2D Thr592) and on the linker between the N-terminal domain and agonist binding domain. CIQ potentiates native NR2D-containing NMDA receptor currents from subthalamic neurons. Our identification of a subunit-selective NMDA receptor modulator reveals a new class of pharmacological tools with which to probe the role of NR2C- and NR2D-containing NMDA receptors in brain function and disease. The involvement of NMDA receptors in neurological diseases including Alzheimer's disease, Parkinson's disease, depression, schizophrenia, epilepsy and injury related to ischaemia, hypoxia or trauma [1] , [2] , [3] , [4] , [5] , [6] , [7] raises the possibility that compounds that potentiate or inhibit NMDA receptor function could have therapeutic benefit [6] , [7] , [8] , [9] , [10] . Compounds that selectively function at one NR2 subunit might modify neuronal function for therapeutic gain only in brain regions in which that subunit is expressed, minimizing side effects due to modulation of other NMDA receptors elsewhere. However, despite decades of work, there is only a single NR2 subunit, NR2B, for which there exist highly (>500-fold) selective pharmacological tools [11] , [12] , [13] . The NR2 subunits show spatially distinct expression patterns throughout the central nervous system. For example, NR2A and NR2B are primarily expressed in rat cortex and hippocampus, whereas the NR2C subunit is highly expressed in cerebellar granule cells, retrosplenial cortex, thalamus, pontine and vestibular nuclei, and oligodendrocytes [14] , [15] , [16] , [17] , [18] , [19] . The NR2D subunit is expressed in deep cerebellar nuclei, subthalamic neurons, striatal neurons and substantia nigra dopaminergic neurons [14] , [15] , [16] , [20] , [21] , [22] , [23] , [24] , [25] . Interestingly, both NR2C and NR2D mRNA are expressed in hippocampal and cortical interneurons [15] , [21] , [22] , [26] , [27] , [28] . The regional and cell-specific expression of the NR2 subunits in the brain coupled with the lack of subunit-selective pharmacological tools motivated us to search for subunit-selective allosteric modulators, which could be useful tools for evaluating the functional role of individual NMDA receptor subunits in normal brain function and in animal models of neurological diseases. We thus evaluated the activity of 100,000 compounds against NR1/NR2C or NR1/NR2D receptors, and identified a class of novel tetrahydroisoquinolines that selectively enhance the responses of NR2C- and NR2D-containing NMDA receptors. 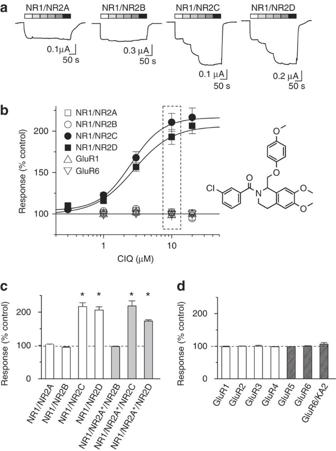Figure 1: CIQ selectively potentiates NR2C and NR2D subunits. (a) Two-electrode voltage-clamp recordings of recombinant NMDA receptors expressed inXenopusoocytes and activated by 100 μM glutamate and 30 μM glycine in the absence and presence of increasing concentrations of CIQ (1–100 μM). (b) Concentration–response curves show the subunit selectivity of CIQ (n=18–21 oocytes per receptor). The response to 100 μM glutamate and 30 μM glycine in the absence of CIQ is normalized to 100%. The structure of CIQ is shown on the right. The dashed box highlights the concentration (10 μM) of CIQ that produces potentiation of responses from NR1/NR2C () and NR1/NR2D () without affecting responses from NR1/NR2A (), NR1/NR2B (), AMPA (GluR1,) and kainate (GluR6,) receptors. (c) The responses of wild-type diheteromeric NMDA receptors to 10 μM CIQ and 100 μM glutamate and 30 μM glycine are shown as a percentage of the response in the absence of CIQ (100%). The responses of NR1/NR2C and NR1/NR2D in the presence of CIQ were significantly different than in control (*P<0.05; pairedt-test;n=6–14). The responses of triheteromeric NMDA receptors containing NR2A(N614K,T690I) (hereafter NR2A*) to 10 μM CIQ in the presence of 10 mM glutamate, 100 μM glycine and 1 mM Mg2+are shown as a percentage of the response in the absence of CIQ (100%). Although triheteromeric receptors composed of NR1/NR2A*/NR2B were not potentiated by CIQ, NR1/NR2A*/NR2C and NR1/NR2A*/NR2D triheteromeric receptors were significantly potentiated by CIQ (*P<0.05; pairedt-test;n=8–18). (d) The responses of GluR1, GluR2, GluR3, GluR4, GluR5 and GluR6 receptors to 100 μM glutamate in the presence of 10 μM CIQ are not significantly different than that in control (n=4–10); oocytes expressing GluR5 and GluR6 were exposed to 10 μM concanavalin A for 10 min before recording. Responses of GluR6/KA2 receptors were evoked by 100 μM AMPA. For all panels, values are mean±s.e.m. Subunit selectivity and mechanism of CIQ Figure 1 shows the structure of (3-chlorophenyl)(6,7-dimethoxy-1-((4-methoxyphenoxy)methyl)-3,4-dihydroisoquinolin-2(1 H)-yl)methanone (CIQ), a chiral compound that emerged from medicinal chemistry efforts to optimize the structure–activity relationship of a single tetrahydroisoquinoline initially identified during screening (see Methods and Supplementary Fig. S1 ). In the presence of both glutamate and glycine, CIQ potentiated the response of rat recombinant NR2C- or NR2D-containing NMDA receptors expressed in Xenopus laevis oocytes in a concentration-dependent manner ( Fig. 1a ). Potentiation was reversible and repeatable. The EC 50 values for potentiation of NR2C- and NR2D-containing receptors were 2.7 and 2.8 μM respectively (maximal potentiation 197±20% and 211±7%; n =21, 18; Fig. 1b ; Supplementary Table S1 ). Similar EC 50 values were found with different NR1 splice variants as well as with human NMDA receptors ( Supplementary Table S2 ). In contrast to its effects on NR1/NR2C and NR1/NR2D receptors, CIQ (10 μM) did not alter recombinant NR1/NR2A, NR1/NR2B, AMPA or kainate receptor responses ( Fig. 1 ). Figure 1: CIQ selectively potentiates NR2C and NR2D subunits. ( a ) Two-electrode voltage-clamp recordings of recombinant NMDA receptors expressed in Xenopus oocytes and activated by 100 μM glutamate and 30 μM glycine in the absence and presence of increasing concentrations of CIQ (1–100 μM). ( b ) Concentration–response curves show the subunit selectivity of CIQ ( n =18–21 oocytes per receptor). The response to 100 μM glutamate and 30 μM glycine in the absence of CIQ is normalized to 100%. The structure of CIQ is shown on the right. The dashed box highlights the concentration (10 μM) of CIQ that produces potentiation of responses from NR1/NR2C ( ) and NR1/NR2D ( ) without affecting responses from NR1/NR2A ( ), NR1/NR2B ( ), AMPA (GluR1, ) and kainate (GluR6, ) receptors. ( c ) The responses of wild-type diheteromeric NMDA receptors to 10 μM CIQ and 100 μM glutamate and 30 μM glycine are shown as a percentage of the response in the absence of CIQ (100%). The responses of NR1/NR2C and NR1/NR2D in the presence of CIQ were significantly different than in control (* P <0.05; paired t -test; n =6–14). The responses of triheteromeric NMDA receptors containing NR2A(N614K,T690I) (hereafter NR2A*) to 10 μM CIQ in the presence of 10 mM glutamate, 100 μM glycine and 1 mM Mg 2+ are shown as a percentage of the response in the absence of CIQ (100%). Although triheteromeric receptors composed of NR1/NR2A*/NR2B were not potentiated by CIQ, NR1/NR2A*/NR2C and NR1/NR2A*/NR2D triheteromeric receptors were significantly potentiated by CIQ (* P <0.05; paired t -test; n =8–18). ( d ) The responses of GluR1, GluR2, GluR3, GluR4, GluR5 and GluR6 receptors to 100 μM glutamate in the presence of 10 μM CIQ are not significantly different than that in control ( n =4–10); oocytes expressing GluR5 and GluR6 were exposed to 10 μM concanavalin A for 10 min before recording. Responses of GluR6/KA2 receptors were evoked by 100 μM AMPA. For all panels, values are mean±s.e.m. Full size image To test whether CIQ could potentiate triheteromeric NMDA receptors containing one NR2C or NR2D subunit, we co-injected oocytes with NR1, NR2C or NR2D, and the magnesium-insensitive, low-glutamate-potency mutant NR2A(N614K, T690I) (hereafter denoted NR2A*) [29] . Oocytes co-injected with NR2A* showed reduced Mg 2+ sensitivity ( Supplementary Fig. S2a ). Moreover, the residual current recorded in the presence of 1 mM Mg 2+ at a holding potential of −80 mV increased with increasing glutamate concentrations only for receptors in oocytes co-injected with NR1, NR2A*, NR2C or NR1, NR2A*, NR2D cRNAs ( Supplementary Fig. S2b ). This suggests that higher glutamate concentrations can activate magnesium-insensitive NR2A*-containing receptors that could be either diheteromeric NR1/NR2A* or triheteromeric receptors containing one NR2A* subunit and one NR2C or NR2D. NR1/NR2C and NR1/NR2D receptors are saturated at all concentrations of glutamate tested (0.1–10 mM), and thus their contribution to the response does not change with increasing concentrations of glutamate. CIQ significantly potentiated the current response recorded in the presence of Mg 2+ from oocytes co-injected with NR1, NR2A*, NR2C or NR1, NR2A*, NR2D cRNA ( Fig. 1c ), but to a lesser extent than NR1/NR2C and NR1/NR2D receptors recorded under identical conditions ( Supplementary Fig. S3 ). Because Mg 2+ did not completely inhibit NR1/NR2C or NR1/NR2D receptors ( Supplementary Fig. S2a ), the intermediate level of CIQ potentiation could be explained if no triheteromeric receptors formed and CIQ simply potentiated the residual NR1/NR2C or NR1/NR2D current (NR1/NR2A* receptors are not potentiated by CIQ; Supplementary Fig. S3 ). However, the level of CIQ potentiation observed in oocytes injected with NR1, NR2A*, NR2C cRNA or NR1, NR2A*, and NR2D cRNA was significantly greater ( P <0.05, Student's t -test; Supplementary Fig. S3 ) than the level of potentiation predicted if no triheteromeric receptors were present (see Methods), suggesting triheteromeric NR1/NR2A*/NR2C and NR1/NR2A*/NR2D receptors were present and were potentiated by CIQ. CIQ potentiation of triheteromeric receptors ( Fig. 1c ) implies that a single NR2C or NR2D subunit was sufficient to confer sensitivity to CIQ. CIQ had no effect on responses of NR1/NR2A*/NR2B receptors ( Fig. 1c ), and no effect on the properties of oocytes injected with cRNA for NR1, NR2A or NR2B alone ( n =5). CIQ did not potentiate recombinant NR1/NR2A ( n =6) and NR1/NR2B receptors ( n =6) expressed in oocytes and activated by the partial agonist NMDA (100 μM) and glycine (30 μM). However, CIQ potentiated recombinant NR1/NR2C ( n =6) and NR1/NR2D receptors ( n =5) activated by 100 μM NMDA and 30 μM glycine (233±13%, 205±5%) to the same extent as responses activated by glutamate ( P =0.75, 0.70, unpaired t -test) with similar EC 50 values (2.7 and 3.3 μM). Thus, the actions of CIQ do not depend on the agonist used to activate the receptor. At peak potentiation, CIQ caused virtually no shift in the EC 50 values for activation of NR1/NR2C or NR1/NR2D receptors by glutamate or glycine ( Table 1 ). Importantly, CIQ alone had no effect on oocytes expressing NR1/NR2C ( n =4) or NR1/NR2D receptors ( n =4) or on uninjected oocytes ( n =4). CIQ also did not activate the receptor in the presence of only glycine ( n =4) or glutamate ( n =4), suggesting that it does not function as an agonist. CIQ potentiated responses in the presence of extracellular Mg 2+ without significantly altering the IC 50 values for Mg 2+ inhibition ( Supplementary Table S1 ). Moreover, CIQ potentiation was not altered at acidic pH values, suggesting CIQ did not relieve tonic proton inhibition ( Supplementary Table S1 ), as proposed for spermine potentiation of NR2B-containing receptors [30] . The potentiating actions of CIQ appeared voltage-independent, with similar degrees of potentiation for both inward and outward currents ( Supplementary Table S3 ). These data suggest that CIQ binding is not allosterically coupled to agonist binding and does not exert its effects through alteration of permeation properties. Table 1 CIQ has minimal effects on glutamate or glycine EC 50 . Full size table CIQ also potentiated current responses of NR2C- and NR2D-containing NMDA receptors expressed in HEK 293 cells at room temperature (23°C) and at 33°C ( Fig. 2 ). Maximal potentiation was 180% for both NR1/NR2C and NR1/NR2D with EC 50 values of 1.7 and 4.1 μM respectively. The time course for the onset of potentiating effects of CIQ was exponential and required several seconds to reach a steady state ( Fig. 2c ). The potentiation by CIQ was rapidly reversible with a time course of de-potentiation that could be fitted by a single exponential component (NR1/NR2C τ 4.0±0.7 s and NR1/NR2D τ 6.5±0.7 s; n =3 and 6). The de-potentiation time constant was independent of CIQ concentration ( Fig. 2d ). The 10–90% rise time of receptor response was rapid in the absence of CIQ (NR2C 6±1 ms; NR2D 13±1 ms) and following pre-application of CIQ (NR2C 9±1 ms; NR2D 15±2 ms), suggesting that CIQ does not require channel opening before binding. 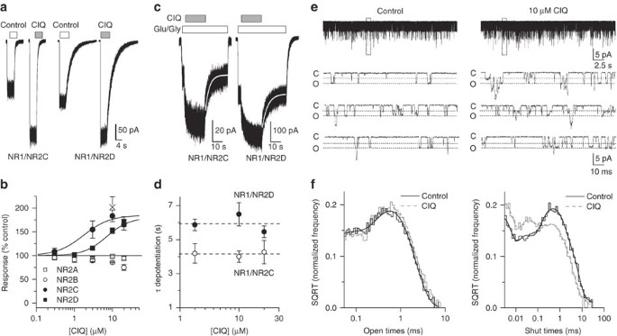Figure 2: CIQ selectively potentiates NR1/NR2C and NR1/NR2D receptors in HEK 293 cells. (a) Representative whole-cell voltage-clamp recordings of NR1/NR2C and NR1/NR2D at 23°C. CIQ (10 μM in 100 μM glutamate and 30 μM glycine) evokes 180% responses from both NR1/NR2C and NR1/NR2D compared with control (100 μM glutamate and 30 μM glycine). (b) The concentration–effect relationships show that CIQ selectively potentiates NR1/NR2C (, EC50=1.7 μM;n=5–11) and NR1/NR2D (, EC50=4.1 μM;n=4–17) to 180% in mammalian cells, but has no effect on NR1/NR2A (,n=4–15). CIQ causes a modest (25%) reduction in the NR1/NR2B response at 20 μM (,n=5). CIQ (10 μM) potentiated the response of NR1/NR2D to NMDA at 33°C by 200±20% (n=5, × on plot). Values are mean±s.e.m. (c) Current responses of NR1/NR2C () and NR1/NR2D () receptors to 100 μM glutamate and 30 μM glycine (white bar) and concurrent application of 10 μM CIQ (grey bar) show that the de-potentiation time course is described by a single exponential function (white line; ref.33). (d) The de-potentiation time course is independent of CIQ concentration for NR1/NR2C (n=3) and NR1/NR2D receptors (n=6). Values are mean±s.e.m. (e) Unitary currents from a representative outside-out patch containing NR1/NR2D receptors activated by 1 mM glutamate and 50 μM glycine in the absence or presence of 10 μM CIQ. The boxed region is expanded below;cdenotes the closed andothe open level. (f) Composite distributions of the contiguous open period durations from six patches can be fitted by two exponential components with time constants of 0.044 and 0.57 ms for control and 0.036 and 0.63 ms for CIQ (see alsoTable 1). The composite closed duration histogram constructed from recordings in the same six patches can be fitted by the sum of six exponential components, with time constants (area in parentheses) of 0.022 (29), 0.19 (14), 1.7 (12), 5.5 (27), 19 (17) and 94 (0.4) ms in the absence and 0.026 (37), 0.23 (18), 0.73 (12), 3.4 (18), 12 (15) and 39 (0.75) ms in the presence of 10 μM CIQ. CIQ (10 μM) had minimal effects on the NMDA receptor deactivation time course ( Table 2 ). Figure 2: CIQ selectively potentiates NR1/NR2C and NR1/NR2D receptors in HEK 293 cells. ( a ) Representative whole-cell voltage-clamp recordings of NR1/NR2C and NR1/NR2D at 23°C. CIQ (10 μM in 100 μM glutamate and 30 μM glycine) evokes 180% responses from both NR1/NR2C and NR1/NR2D compared with control (100 μM glutamate and 30 μM glycine). ( b ) The concentration–effect relationships show that CIQ selectively potentiates NR1/NR2C ( , EC 50 =1.7 μM; n =5–11) and NR1/NR2D ( , EC 50 =4.1 μM; n =4–17) to 180% in mammalian cells, but has no effect on NR1/NR2A ( , n =4–15). CIQ causes a modest (25%) reduction in the NR1/NR2B response at 20 μM ( , n =5). CIQ (10 μM) potentiated the response of NR1/NR2D to NMDA at 33°C by 200±20% ( n =5, × on plot). Values are mean±s.e.m. ( c ) Current responses of NR1/NR2C ( ) and NR1/NR2D ( ) receptors to 100 μM glutamate and 30 μM glycine (white bar) and concurrent application of 10 μM CIQ (grey bar) show that the de-potentiation time course is described by a single exponential function (white line; ref. 33 ). ( d ) The de-potentiation time course is independent of CIQ concentration for NR1/NR2C ( n =3) and NR1/NR2D receptors ( n =6). Values are mean±s.e.m. ( e ) Unitary currents from a representative outside-out patch containing NR1/NR2D receptors activated by 1 mM glutamate and 50 μM glycine in the absence or presence of 10 μM CIQ. The boxed region is expanded below; c denotes the closed and o the open level. ( f ) Composite distributions of the contiguous open period durations from six patches can be fitted by two exponential components with time constants of 0.044 and 0.57 ms for control and 0.036 and 0.63 ms for CIQ (see also Table 1 ). The composite closed duration histogram constructed from recordings in the same six patches can be fitted by the sum of six exponential components, with time constants (area in parentheses) of 0.022 (29), 0.19 (14), 1.7 (12), 5.5 (27), 19 (17) and 94 (0.4) ms in the absence and 0.026 (37), 0.23 (18), 0.73 (12), 3.4 (18), 12 (15) and 39 (0.75) ms in the presence of 10 μM CIQ. Full size image Table 2 CIQ has minimal effects on NMDA receptor deactivation. Full size table Single-channel analysis of CIQ To determine the mechanism by which CIQ enhanced the NMDA receptor response, the actions of CIQ on NMDA receptor single-channel properties were examined. Application of 1 mM glutamate and 50 μM glycine to excised outside-out patches containing rat recombinant NR1/NR2D receptors produced unitary currents with properties similar to those previously described [31] , [32] . Unitary currents showed two sublevels with chord conductance values of 33 and 56 pS in 0.5 mM extracellular Ca 2+ . Co-application of 10 μM CIQ increased the open probability to 190±25% of control ( n =11) in a reversible manner ( Fig. 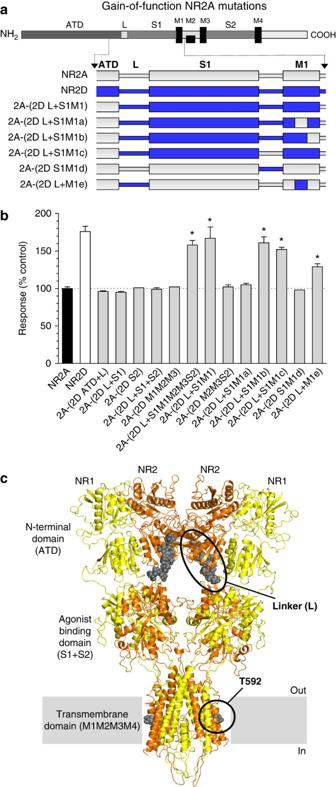Figure 3: Structural determinants for transferring CIQ sensitivity to NR2A. (a) Schematic representation of the NR2 subunit polypeptide illustrates regions comprising the N-terminal domain (ATD), the agonist binding domain (two segments of the polypeptide chain called S1 and S2), a membrane-associated domain that forms the ion channel pore and contains three membrane-spanning helices (M1, M3 and M4) with a re-entrant loop (M2), and an intracellular C-terminal domain. Schematic representations of chimeras between the NR2D ATD-M1 region and the corresponding region in NR2A are shown (seeSupplementary Table S4for chimeric junctions). Regions from NR2A and NR2D are shown in light grey and dark solid blue respectively. (b) The response to 10 μM CIQ and 100 μM glutamate and 30 μM glycine is shown as a percentage of the response in the absence of CIQ. CIQ sensitivity is observed (*P<0.05 compared with wild-type NR2A; one-way analysis of variance with Dunnett's post test) for chimeras 2A-(2D L+S1M1M2M3S2), 2A-(2D L+S1M1), 2A-(2D L+S1M1b), 2A-(2D L+S1M1c) and 2A-(2D L+M1e), suggesting that transfer of CIQ sensitivity to NR2A requires residues 590–594 from NR2D and the NR2D linker region (L) between the ATD and the S1 region. Results are from 4–23 oocytes per receptor tested. Values are mean±s.e.m. (c) Model of an NR1/NR2 heterodimer of the tetrameric NMDA receptor based on the GluR2 structure34is shown. M4 and the C-terminal domain are omitted for clarity. The NR1 and NR2 subunits are shown in yellow and brown respectively. The regions that together can transfer CIQ sensitivity from NR2D to NR2A (T592 and the ATD-S1 linker) are shown as grey spheres and highlighted in black circles. 2e ; Table 3 ). The effect of CIQ on open probability is solely due to an effect on mean shut time ( Fig. 2f ), as CIQ decreased mean shut time to 75±8% of control ( n =11). The mean open time was unchanged by CIQ, as were individual fitted exponential components describing the open duration histogram ( Fig. 2f , Table 3 ). CIQ had minimal effects on chord conductance and no detectable effect on the reversal potential. CIQ had no significant effect on the relative frequency of the lower conductance level and did not alter relative frequency of direct 33–56 pS or 56–33 pS sublevel transitions. These data suggest that CIQ binds to a site on the NMDA receptor that influences channel opening, without altering the stability of the open state or the nature of the permeation pathway. We interpret these data to suggest that CIQ likely functions to facilitate pregating steps that follow agonist binding and either precede or are involved in pore dilation. Table 3 NR1/NR2D channel properties in the presence of CIQ. Full size table Molecular determinants of CIQ To identify the molecular determinants of CIQ activity, we measured responses of NMDA receptors containing NR2A-NR2D chimeric subunits ( Fig. 3 ; see Supplementary Fig. S4 and Supplementary Table S4 for chimeric junctions). Taking advantage of the fact that CIQ potentiates NR1/NR2D receptors but not NR1/NR2A receptors, we first evaluated the portions of NR2D that, when inserted into NR2A, transferred CIQ sensitivity. Evaluation of these chimeric receptors for a gain of function suggested that the molecular determinants of CIQ selectivity for NR2D over NR2A reside in the L–S1–M1 region ( Fig. 3a and b ). Further assessment of chimeric receptors containing progressively smaller portions of the NR2D subunit narrowed down the regions of interest to the linker (L) between the ATD and ligand binding domain plus five residues (590–594) in the M1 transmembrane helix of NR2D. The chimera NR2A-(2D L+M1e) containing only these two regions from NR2D was potentiated by 10 μM CIQ ( Fig. 3b ). CIQ did not show any activity when the ATD-S1 linker (L) of NR2D alone was transferred to NR2A ( n =16), or when residues 590–594 in NR2D alone were transferred to NR2A ( n =4) ( Supplementary Table S4 ). The open probability of NR1/NR2D (0.01) is lower than that of NR1/NR2A (0.5) [33] , raising the possibility that CIQ facilitation of channel opening might require a low open probability. Consistent with this idea, the ATD-S1 linker (L) between the ATD and ligand binding domain of NR2D has previously been shown to reduce open probability when introduced into NR2A [33] . Figure 3: Structural determinants for transferring CIQ sensitivity to NR2A. ( a ) Schematic representation of the NR2 subunit polypeptide illustrates regions comprising the N-terminal domain (ATD), the agonist binding domain (two segments of the polypeptide chain called S1 and S2), a membrane-associated domain that forms the ion channel pore and contains three membrane-spanning helices (M1, M3 and M4) with a re-entrant loop (M2), and an intracellular C-terminal domain. Schematic representations of chimeras between the NR2D ATD-M1 region and the corresponding region in NR2A are shown (see Supplementary Table S4 for chimeric junctions). Regions from NR2A and NR2D are shown in light grey and dark solid blue respectively. ( b ) The response to 10 μM CIQ and 100 μM glutamate and 30 μM glycine is shown as a percentage of the response in the absence of CIQ. CIQ sensitivity is observed (* P <0.05 compared with wild-type NR2A; one-way analysis of variance with Dunnett's post test) for chimeras 2A-(2D L+S1M1M2M3S2), 2A-(2D L+S1M1), 2A-(2D L+S1M1b), 2A-(2D L+S1M1c) and 2A-(2D L+M1e), suggesting that transfer of CIQ sensitivity to NR2A requires residues 590–594 from NR2D and the NR2D linker region (L) between the ATD and the S1 region. Results are from 4–23 oocytes per receptor tested. Values are mean±s.e.m. ( c ) Model of an NR1/NR2 heterodimer of the tetrameric NMDA receptor based on the GluR2 structure [34] is shown. M4 and the C-terminal domain are omitted for clarity. The NR1 and NR2 subunits are shown in yellow and brown respectively. The regions that together can transfer CIQ sensitivity from NR2D to NR2A (T592 and the ATD-S1 linker) are shown as grey spheres and highlighted in black circles. Full size image To identify the elements required for CIQ potentiation of NR2D, we evaluated a series of NR2D mutations for loss of function. Insertion of the NR2A ATD-S1 linker (L) into NR2D did not significantly alter CIQ potentiation (2D-(2A L); Fig. 4 ). CIQ potentiation of chimeric receptors in which both the NR2A ATD and ATD-S1 linker (2D-(2A ATD+L)) are placed into NR2D is attenuated ( Fig. 4b ). This result is consistent with the idea that some elements of the ATD beyond the linker enhance the actions of CIQ on NR2D. Site-directed mutagenesis within the M1 region of NR2D identified a single residue (Thr592) that is conserved in NR2C/D but different in NR2A/B as an important determinant of activity ( Fig. 4b ). In contrast to results with NR2D-(NR2A L) chimeric receptors, mutagenesis of this residue to the corresponding residue in NR2A (NR2D T592I) completely abolished the potentiating actions of CIQ ( Fig. 4b ). CIQ (10 μM) significantly potentiated NR2A-containing receptors with the corresponding reverse mutation NR2A(I567T) and the linker (L) between NR2D ATD and S1 (135±5%, n =12). However, this point mutation in NR2A (I567T), along with the NR2D ATD-S1 linker, was not sufficient to transfer the full CIQ potentiation observed at NR1/NR2D to NR1/NR2A (see Supplementary Table S4 ). These data show consistent gain-of-function and loss-of-function effects relating to residue Thr592 in the NR2D M1 region ( Fig. 3c ). These data also identify the ATD and linker between ATD and S1, which has divergent sequences across all four NR2 subunits, as an important structural determinant of CIQ actions in NR2D ( Fig. 3c ). 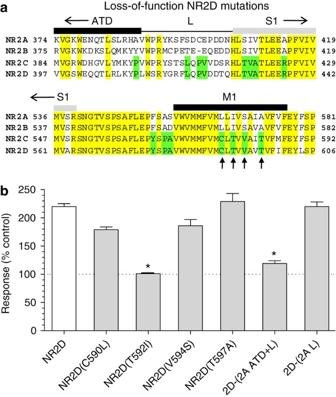Figure 4: Structural determinants of CIQ action in NR2D. (a) Alignment of amino-acid sequences for the ATD-S1 linker and M1 regions of NR2A-D. Fully conserved residues are shown in yellow, and residues conserved only in NR2C and NR2D are shown in green. Arrows mark residues that were converted in NR2D from the NR2C/D residue to the NR2A/B residue andvice versaby site-directed mutagenesis (Supplementary Table S4). (b) Four M1 residues in NR2D that are conserved between NR2C/D but not NR2A/B were mutated to the corresponding residue in NR2A/B. Responses of the mutant receptor NR1/NR2D(T592I) were no longer potentiated by CIQ. Chimeric NR2D receptors with the ATD+L showed a reduced level of potentiation. Results are from 6–10 oocytes per receptor tested (*P<0.05 compared with NR1/NR2D, one-way analysis of variance with a Tukey'spost hoctest). Values are mean±s.e.m. Figure 4: Structural determinants of CIQ action in NR2D. ( a ) Alignment of amino-acid sequences for the ATD-S1 linker and M1 regions of NR2A-D. Fully conserved residues are shown in yellow, and residues conserved only in NR2C and NR2D are shown in green. Arrows mark residues that were converted in NR2D from the NR2C/D residue to the NR2A/B residue and vice versa by site-directed mutagenesis ( Supplementary Table S4 ). ( b ) Four M1 residues in NR2D that are conserved between NR2C/D but not NR2A/B were mutated to the corresponding residue in NR2A/B. Responses of the mutant receptor NR1/NR2D(T592I) were no longer potentiated by CIQ. Chimeric NR2D receptors with the ATD+L showed a reduced level of potentiation. Results are from 6–10 oocytes per receptor tested (* P <0.05 compared with NR1/NR2D, one-way analysis of variance with a Tukey's post hoc test). Values are mean±s.e.m. Full size image Actions of CIQ on native NMDA receptors The NR2D subunit has been suggested to be the predominant NMDA receptor NR2 subunit expressed in neurons of the subthalamic nuclei [20] . We therefore evaluated the ability of CIQ to potentiate native NMDA receptor responses in subthalamic neurons using whole-cell voltage-clamp recordings of current responses to pressure application of NMDA and glycine in the absence of synaptic transmission. This approach provides tight control over the amount of agonist released, which activates both synaptic and extra-synaptic receptors ( Fig. 5a ). NMDA receptor responses were produced by pressure release of agonist at 1 min intervals in neurons held at −60 mV and bathed in artificial cerebrospinal fluid (ACSF) containing 0.2 mM Mg 2+ , 0.5 μM TTX, 5 μM nimodipine and 10 μM bicuculline. NMDA receptor responses were evaluated before, during and after bath application of CIQ (20 μM). CIQ potentiated NMDA-activated responses in six out of six subthalamic neurons by an average of 230±29% ( n =6; Fig. 5b , white bars, c). Potentiation by CIQ was reversible; responses after wash were not significantly different than control responses (102±11%; n =6; Fig. 5b and c ). Application of vehicle alone had no significant effect on response amplitude to pressure-applied NMDA and glycine (106±9%, n =5; P =0.25). NMDA-activated responses could be largely inhibited by bath application of 200–400 μM of the competitive NMDA receptor antagonist D,L-APV. CIQ did not potentiate NMDA-activated responses of CA1 hippocampal pyramidal neurons ( n =5; Fig. 5b , grey bars, d), which have been shown to express predominantly NR2A and NR2B NMDA receptor subunits [15] , showing that potentiation by CIQ is selective for native NR2C/D-containing NMDA receptors. 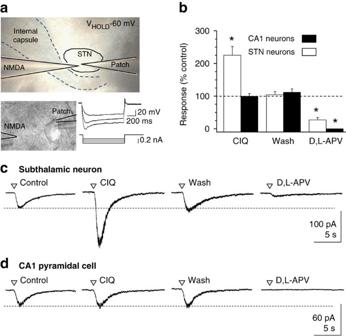Figure 5: CIQ potentiates native NR2D-containing NMDA receptors in subthalamic neurons. (a) Photomicrograph of the experimental setup for whole-cell voltage-clamp recording from subthalamic (STN) neurons. A pressurized (4–12 p.s.i.; 3–100 ms application) micropipette (3.5 MΩ) was used to apply glycine (0.5–1 mM) and NMDA (1–2 mM) to the subthalamic neuron, which was held at −60 mV. Lower right, neurons demonstrated characteristicIhcurrent, evoked by injecting 0.1 nA hyperpolarizing current into the cell. (b) CIQ (20 μM) potentiated STN neurons to 230±29% (n=6; white bars) compared with the control response. Potentiation by CIQ was reversible, with NMDA-activated responses after recovery being 102±11% of control amplitude. NMDA-activated responses could be inhibited by the NMDA receptor competitive antagonist D,L-APV (200–400 μM; 27±7% residual current compared with control). CIQ did not potentiate the current response to pressure-applied NMDA in hippocampal CA1 pyramidal neurons (n=5; black bars). Data are mean±s.e.m. *P<0.01; one-way repeated-measures analysis of variance and Tukey'spost hoctest. (c) Representative whole-cell voltage-clamp recordings of the current response to pressure-applied NMDA/glycine in a subthalamic neuron show that CIQ potentiation was reversible, and that NMDA-evoked currents were inhibited by D,L-APV. (d) Representative whole-cell voltage-clamp recording from a hippocampal CA1 pyramidal neuron in response to pressure-applied NMDA and glycine shows that CIQ potentiation is selective for NR2C/D-containing receptors over NR2A/B-containing receptors. Figure 5: CIQ potentiates native NR2D-containing NMDA receptors in subthalamic neurons. ( a ) Photomicrograph of the experimental setup for whole-cell voltage-clamp recording from subthalamic (STN) neurons. A pressurized (4–12 p.s.i. ; 3–100 ms application) micropipette (3.5 MΩ) was used to apply glycine (0.5–1 mM) and NMDA (1–2 mM) to the subthalamic neuron, which was held at −60 mV. Lower right, neurons demonstrated characteristic I h current, evoked by injecting 0.1 nA hyperpolarizing current into the cell. ( b ) CIQ (20 μM) potentiated STN neurons to 230±29% ( n =6; white bars) compared with the control response. Potentiation by CIQ was reversible, with NMDA-activated responses after recovery being 102±11% of control amplitude. NMDA-activated responses could be inhibited by the NMDA receptor competitive antagonist D,L-APV (200–400 μM; 27±7% residual current compared with control). CIQ did not potentiate the current response to pressure-applied NMDA in hippocampal CA1 pyramidal neurons ( n =5; black bars). Data are mean±s.e.m. * P <0.01; one-way repeated-measures analysis of variance and Tukey's post hoc test. ( c ) Representative whole-cell voltage-clamp recordings of the current response to pressure-applied NMDA/glycine in a subthalamic neuron show that CIQ potentiation was reversible, and that NMDA-evoked currents were inhibited by D,L-APV. ( d ) Representative whole-cell voltage-clamp recording from a hippocampal CA1 pyramidal neuron in response to pressure-applied NMDA and glycine shows that CIQ potentiation is selective for NR2C/D-containing receptors over NR2A/B-containing receptors. Full size image The physiological, pharmacological and biophysical properties of NMDA receptors are governed by the NR2 subunit [1] . Despite the important role of NMDA receptors in central nervous system function and neurological disorders, there remains a surprising lack of molecules that function on NMDA receptors with sufficient subunit selectivity to allow evaluation of the role of NR2 subunits in normal function and disease. We report here the first drug-like NMDA receptor-positive allosteric modulator (CIQ) that potentiates NR2C- and NR2D-containing NMDA receptor responses with strong subunit selectivity. Although the data do not unequivocally identify a binding site for CIQ, molecular studies reveal structural determinants of subunit selectivity, and support the idea that CIQ binds to a new modulatory site that is either near the NR2 M1 region or near NR2 ATD and associated linker. Mechanistic studies suggest that CIQ binding reduces the activation energy for key conformational changes that lead to channel opening, without altering the stability of the open state. Studies of native receptors in the absence of synaptic transmission show that CIQ can potentiate NMDA receptor responses of subthalamic neurons to exogenously applied NMDA. Thus, CIQ represents a new class of subunit-selective NMDA receptor modulators with which to probe the role of NR2C- and NR2D-containing NMDA receptors in brain function and disease. Two-electrode voltage-clamp recordings from X. laevis All procedures involving the use of animals were reviewed and approved by the Emory University IACUC. Oocytes from X. laevis were isolated, injected with cRNA synthesized in vitro and recorded under voltage-clamp as previously described [35] . The recording solution contained (in mM) 90 NaCl, 3 KCl, 10 HEPES, 0.01 EDTA, 0.5 BaCl 2 (23°C); pH was adjusted to 7.4 with NaOH. Glutamate-evoked membrane currents (50–100 μM) were recorded at −40 mV in the presence of 30–100 μM glycine 24–72 h after injection unless otherwise indicated. Triheteromeric NMDA receptors consist of NR1 and two NR2 subunits were studied using the method of Hatton and Paoletti [29] . Briefly, NR2B, NR2C or NR2D cRNA was co-injected with cRNA encoding NR2A(N614K,T690I) (referred to as NR2A*) and NR1 at a ratio of 1:3:2 (20 ng total). Responses to glutamate (10 mM) and glycine (100 μM) were recorded at −80 mV 24–72 h after injection. NR1/NR2A* receptors were insensitive to block by Mg 2+ and had reduced glutamate potency. Thus, NR2A* should allow isolation of triheteromeric receptors when co-expressed with NR1 and NR2B, NR2C or NR2D by recording in the presence of 1 mM Mg 2+ and 10 mM glutamate [29] . We estimated the maximum possible level of potentiation solely due to NR1/NR2C receptors in the residual response. If one assumes that no triheteromeric receptors were present in oocytes injected with NR1, NR2A*, NR2C cRNA, then the relative current in Mg 2 would be solely due to NR1/NR2C and NR1/NR2A* receptors, with the relative contribution determined by where α is the fraction of the current from NR1/NR2C receptors, β the fraction of current from NR1/NR2A* receptors and ( I Mg / I Control ) is the residual current response in the presence of 1-mM Mg 2+ at −80 mV ( Supplementary Fig. S2a ). Assuming no triheteromeric receptors were formed, we can calculate α =0.813 and β =0.187 from this equation for NR2C using the data shown in Supplementary Figure S2a . Because CIQ has no detectable effect on NR1/NR2A* receptors ( Supplementary Fig. S3a ), we can calculate the maximum possible CIQ potentiation solely due to residual NR1/NR2C according to the equation where I CIQ / I Control is the ratio of current in the presence of CIQ to that in the absence of CIQ at NR1/NR2C receptors (2.7) under these recording conditions ( Supplementary Fig. S3 ). Similar calculations have been made for NR1/NR2D ( Supplementary Figs S2 and S3 ). Patch-clamp recording from HEK 293 cells HEK 293 cells were maintained in 5% humidified CO 2 at 37°C in DMEM (Invitrogen) supplemented with 10% fetal bovine serum, 10 U ml −1 penicillin and 10 μg ml −1 streptomycin and were transiently transfected using the Fugene 6 transfection reagent with cDNAs encoding NMDA receptor subunits and green fluorescent protein (GFP) at a ratio (NR1/NR2/GFP) of 1:1:1 or 1:1:5 (2 μg total DNA) for 12–16 h [36] . Current responses from voltage-clamp recordings of HEK cells ( V HOLD =−60 mV) and outside-out patches ( V HOLD =−80 mV) were filtered at 8 kHz (8 pole Bessel filter, −3 dB) and digitized at 20–40 kHz. The extracellular solution consisted of (in mM) 150 NaCl, 10 HEPES, 0.5 CaCl 2 , 3 KCl, 0.01 EDTA and 30 D -mannitol (pH 7.4). The internal solution consisted of (in mM) 110 D -gluconate, 110 CsOH, 30 CsCl 2 , 5 HEPES, 4 NaCl, 0.5 CaCl 2 , 2 MgCl 2 , 5 BAPTA, 2 NaATP and 0.3 NaGTP (pH adjusted to 7.35 with CsOH). For whole-cell patch recordings, rapid solution exchange was achieved with a two-barrel theta glass pipette controlled by a piezoelectric translator. Open tip junction currents typically had 10–90% rise times of 1 ms or less; solution exchange around a whole cell was determined by changing the concentration of extracellular potassium, which altered the leak current with a 10–90% rise time of 5 ms [37] . Single-channel recordings from outside-out patches were taken at pH 8.0 using steady-state application of agonist. All recordings were performed at 23°C unless otherwise indicated. Patch-clamp recording from neurons in thin slices Rats (Sprague–Dawley, age P10–P17) were anaesthetized using isoflurane, decapitated, and the brain was hemisected and glued to the stage of a vibrating microtome (Leica VT1000S). Sagittal brain slices were cut in cold ACSF composed of (in mM) 130 NaCl, 24 NaHCO 3 , 10 glucose, 3 KCl, 3 MgSO 4 , 1.25 NaH 2 PO 4 and 1 CaCl 2 , and incubated at room temperature in the same solution for at least 1 h before use. Slices containing the subthalamic nucleus or hippocampus were placed in the recording chamber of an upright microscope for whole-cell voltage-clamp recordings. Slices were perfused with ACSF composed of (in mM) 130 NaCl, 24 NaHCO 3 , 10 glucose, 3 KCl, 1.5 MgSO 4 , 1.5 CaCl 2 and 1.25 NaH 2 PO 4 saturated with 95%O 2 /5% CO 2 at pH 7.4 (23°C). Voltage-clamp recordings were taken at −60 mV, filtered at 5 kHz and digitized at 20 kHz. Patch recording electrodes were filled with (in mM) 115 K-methylsulphate, 20 NaCl, 10 phosphocreatine, 5 HEPES, 2 Mg-ATP, 1.5 MgCl 2 , 1 QX-314, 0.5 Na-GTP and 0.1 EGTA at pH 7.5. Recording solutions contained 0.2 mM MgSO 4 , 0.5 μM TTX, 10 μM bicuculline and 5 μM nimodipine. Currents were evoked when NMDA (1–2 mM) and glycine (0.5–1 mM) were pressure applied through a borosilicate capillary tube (3.5 MΩ) in brief pulses (4–12 p.s.i. ; 3–100 ms) using a Picospritzer II (Parker Hannifin). After 3–10 stable measurements were obtained in the presence of the control solution at 1 min intervals, CIQ (20 μM, prepared in recording solution) or vehicle was bath applied for 10–15 min. Current responses evoked by pressure application of NMDA and glycine were compared with currents obtained during application of control ACSF. Following bath application of CIQ, the slice was washed with the control recording solution and NMDA and glycine continued to be pressure applied at a 1 min interval to determine the degree of CIQ washout. The NMDA receptor competitive antagonist D,L-APV (200–400 μM) was subsequently bath applied during NMDA and glycine applications. The I h current was recorded under current-clamp using the same intracellular solution by injecting 0.1 nA of current into the cell. Synthesis and physicochemical properties of CIQ CIQ (C 26 H 26 ClNO 5 ; molecular weight 467.94) was synthesized from commercially available starting materials (see Supplementary Methods and Supplementary Fig. S1 ). CIQ is also commercially available and can be obtained from Life Chemicals (catalogue no. F0535-0139). Characterization and determination of purity were established by 1 H NMR, 13 C NMR, high-resolution mass spectrometry and elemental combustion analysis. All experiments were conducted on the racemic mixture. CIQ has a predicted log P -value of 4.95 from ChemDraw. The total polar surface area (that is, van der Waals surface area of polar nitrogen and oxygen atoms) is 58.5 Å [2] . The maximum solubility of CIQ was determined using a BMG Labtech Nephelostar nephelometer (Offenburg) according to the manufacturer's instructions, and was 20 μM. CIQ did not form detectable micelles at 10 μM when dissolved in HEK 293 extracellular recording solution or in filtered H 2 O, as assessed using a Zetasizer dynamic light scattering instrument (Malvern Instruments). No detectable micelles or nanoparticles were observed during examination of evaporated solution with a Hitachi H-7500 transmission electron microscope (accelerated voltage 75 kV; magnifications from ×5 to ×100K). CIQ was dissolved in 100% dimethylsulphoxide (DMSO) to prepare 200–2000× stock solutions that were then added directly to oocyte recording solutions to give a final solution containing a maximum of 0.05–0.5% DMSO. All recordings from mammalian cells used 1:1000–1:2000 dilution of 20 mM stock (0.05–0.1% DMSO). DMSO was not required for activity, as CIQ dissolved in 2-hydroxypropyl-β-cyclodextrin solution (1%, w/v) potentiated NR1/NR2D receptor responses in oocytes (144±3% of control; n =4). DMSO did not induce any potentiation of NR1/NR2D responses in oocytes (100±1.1% of control; n =6) or HEK cells (106±7.7, n =3). Molecular biology The following constructs encoding wild-type NMDA receptor subunits were used: rat NR1-1a and all other rat NR1 splice variants (GenBank U11418, U08261; hereafter NR1), rat NR2A (D13211), rat NR2B (U11419), rat NR2C (M91563) and rat NR2D (L31611), modified as described [15] . Chimeric NR2 subunits containing portions of rat NR2A and NR2D were generated as previously described [38] using PCR strategies and verified by DNA sequencing. Detailed information about the NR2A-NR2D chimeric junctions is summarized in Supplementary Figure S4 . Amino acids are numbered according to full-length protein, including the signal peptide. Data analysis Single-channel recordings from outside-out patches were idealized using the SKM algorithm of QuB [39] ( http://www.qub.buffalo.edu ) for measurement of open probability, mean shut time and opening frequency. Open probability was calculated as the total duration of time that all detected channels in the patch were open divided by the total recording time. Because we cannot be sure of the total number of channels, this measurement does not represent the probability that one channel will open, but rather is the product of the probability that one channel will open and the number of channels in the patch. In a subset of high-quality patches with adequately low noise, segments in which no double openings were observed were idealized using time course fitting (SCAN; provided by Dr David Colquhoun, University College London [40] ) for measurement of individual open and closed durations, mean open time, unitary current amplitudes and chord conductances. Amplitude histograms were fitted by the sum of multiple Gaussian components, and open and closed duration distributions were fitted with the sum of 2–5 exponential functions using maximum likelihood methods [40] . The deactivation time courses of the current responses were fitted by two exponential components using where τ FAST and τ SLOW are the deactivation time constants. The concentration–effect relationships for agonists were fitted to the Hill equation where EC 50 is the concentration of agonist that produces a half-maximally effective response and N the Hill slope. The concentration–effect relationships for CIQ potentiation were fitted to where EC 50 is the concentration of CIQ that produces a half-maximally effective potentiation and N the Hill slope. Statistical analysis Student's paired t -test (two tailed) or analysis of variance (Dunnett's, Tukey's post hoc test) was used for statistical comparisons, as appropriate ( P <0.05 was considered statistically significant). All data are expressed as mean±s.e.m. Although concentration–response EC 50 data are given as mean±s.e.m., statistical tests were performed on the log(EC 50 ), because EC 50 shows a lognormal distribution [41] , [42] . How to cite this article: Mullasseril P, et al . A subunit-selective potentiator of NR2C- and NR2D-containing NMDA receptors. Nat. Commun. 1:90 doi: 10.1038/ncomms1085 (2010).